An authentic imaging probe to track cell fate from beginning to end Accurate tracing of cell viability is critical for optimizing delivery methods and evaluating the efficacy and safety of cell therapeutics. A nanoparticle-based cell tracker is developed to image cell fate from live to dead. The particle is fabricated from two types of optically quenched polyelectrolytes, a life indicator and a death indicator, through electrostatic interactions. On incubation with cells, the fabricated bifunctional nanoprobes are taken up efficiently and the first colour is produced by normal intracellular proteolysis, reflecting the healthy status of the cells. Depending on the number of coated layers, the signal can persist for several replication cycles. However, as the cells begin dying, the second colour appears quickly to reflect the new cell status. Using this chameleon-like cell tracker, live cells can be distinguished from apoptotic and necrotic cells instantly and definitively. Cell therapies, including stem cell therapy, have been considered as alternative approaches for various regenerative diseases; however, initial studies have been disappointing, partially because the distribution and function of the injected cells were unable to be assessed in real time [1] . This limitation made optimization difficult and indirectly contributed to poor therapeutic outcomes. Over the past few decades, imaging technologies and downstream applications have dramatically advanced. Visualizing or tracking biological processes for diagnostic and therapeutic purposes provides critical information in guiding medical research and clinical operations [2] . Similarly, advanced imaging technology that is capable of tracking therapeutic cells could aid the development of cell therapies. Thus far, only a few non-invasive imaging technologies have been developed to monitor distribution, functionality and viability of injected cells [3] , [4] , [5] . To study injected cells, transgenic reporters, such as green fluorescent protein, luciferase and thymidine kinase, have been widely used in animals [6] , [7] . However, introducing a foreign gene into therapeutic cells always causes safety concerns, such as the potential risk of immunogenicity and tumorigenicity induced by random integration of reporter genes [8] , [9] . Compared with a simple chemical labelling approach, transfection procedures are also time consuming. Thus, various synthetic materials have been used as imaging reagents, including organic dyes, polymers and inorganic nanoparticles [10] , [11] , [12] . Although inorganic nanoparticles, such as quantum dots, are highly luminescent and resistant to photobleaching, their usage for cell labelling is limited due to their potential cytotoxicity and unstable fluorescence signals, especially in dividing cells [13] , [14] . Alternatively, fluorescent dyes were developed in parallel to track cells in real time in vivo [15] , [16] . In addition to tracking the distribution of the injected cells, their viability is another critical factor for cell therapy. Methods for non-invasive imaging of cell death (that is, apoptosis and necrosis) have been developed to report cell states and their responses to therapeutic interventions [17] , [18] . Both intracellular biomarkers, such as caspases [19] , [20] and mitochondrial membrane potential [21] , and extracellular biomarkers, such as plasma membrane phosphatidylserine [22] , [23] , [24] , phosphatidylethanolamine [25] and cell surface-exposed histone [26] , are regularly used to indicate apoptosis. For necrosis, the most accepted biomarker is DNA that becomes accessible after disruption of the cell plasma membrane [27] . DNA-binding agents, such as Hoechst [28] and hypericin [29] , are used to label extracellular DNA released from necrotic cells. Although the aforementioned protocols provide valuable information about injected cells, they can only report the current status of the cells when the labelling agent was applied. They are unable to reflect the status of cells over long periods of time. A multifunctional cell tracker, capable of reporting cell fate from live to dead in real time, would be extremely valuable for optimizing cell therapy. Recently, we developed a long-lasting cell tracker containing a fluorescence signal that is able to last more than 3 weeks without noticeable cell toxicity [30] . Based on this live-cell imaging platform, a novel ingredient was included as a cell death reporter. The cell of interest could be conveniently labelled by simply mixing with the synthesized nanoprobe in vitro . The initial intracellular fluorescent colour is stable in healthy cells for long periods of time. Should the cells turn apoptotic or necrotic, the nanoprobe will send a new fluorescence signal, which can be identified clearly by monitoring a second wavelength. Live cell tracker (L 3 ) The previously developed long-lasting probes were assembled by layering fluorochrome decorated poly- L -lysine (PLL) and poly(acrylic acid) (PAA) on an inert gold nanoparticle (AuNP) core, using a layer-by-layer deposition technique [30] , [31] . In living cells, PLL is degraded naturally by several intracellular proteases such as cathepsin B and cathepsin L [32] , [33] . As the number of fluorochromes per PLL molecule was optimized for the maximum quenching of fluorescence at initial state and maximum recovery of fluorescence when it was degraded proteolytically in cells, a high signal-to-background ratio was observed while using this system. It was also confirmed that the nanoprobes, made of protease-resistant poly- D -lysine (PDL) are not activated in cells [30] ; thus, no fluorescence signal could be detected in healthy cells, even after several days of incubation. However, during the studies, a few highly fluorescent round cells that were presumed dead were noticed occasionally. It was suspected that those bright fluorescence signals were generated by PDL degradation in the course of cell death. Based on this interesting observation, we thought that the PDL-containing nanoprobe could be useful in imaging cell death. To prove this hypothesis, PLL with cyanine dye (cy) 5.5 and PDL with fluorescein isothiocyanate (FITC) were prepared for live-cell and dead-cell imaging, respectively. The optimal loading ratio of cy5.5 per PLL molecule was assessed using a series of cy5.5 concentrations, and their protease accessibility was determined using trypsin as a model protease. Cy5.5/PLL ratios were from 1/1 to 7/1, and the optimal ratio was found to be 7/1 (termed PLL-C7) among all preparations. This ratio provided the maximum dequenching value on protease treatment (>9-fold) ( Supplementary Fig. 1 ). The activation of PLL-C6 (6/1 ratio of Cy5.5/PLL) was slightly lower than that of PLL-C7. Nanoprobes, NP-(PLL-C n ) 3 , were then fabricated with three layers of PLL-C n polymers using the previously developed protocol and subjected to protease activation ( Supplementary Fig. 2a ). All of the fabricated nanoprobes were stable in phosphate-buffered saline (PBS), but when treated with trypsin the fluorescence signal increased significantly ( Supplementary Fig. 2b ). The optimal formulations were the ones assembled with PLL-C6 (NP-(PLL-C6) 3 ) and PLL-C7 (NP-(PLL-C7) 3 ), whose fluorescence increased by >250-fold after 24 h of incubation. PLL-C6 was then selected to prepare nanoprobes with three layers of PLL-C6 (termed L 3 ) for subsequent studies. Dead cell tracker (D 3 ) Conversely, PDL was labelled with the same number of FITC molecules (FITC/PDL=6/1) and the nanoprobes were fabricated by coating them with three layers of PDL–FITC (termed D 3 ) using the same protocol. When the formulated nanoprobes were exposed to trypsin in tubes, as expected, fluorescence change was not detected in D 3 , but it increased quickly in L 3 , supporting the hypothesis that normal proteolysis cannot cleave unnatural PDL ( Supplementary Fig. 3 ). To validate the hypothesis that PDL would be cleaved in dying cells, D 3 nanoprobes ( Fig. 1a ) were investigated in both healthy and apoptotic cells. Healthy MDA-MB231 cells were incubated with D 3 and then washed with complete culture medium. A commercially available apoptotic cell-labelling reagent, Annexin V-cy3, was added to detect apoptotic cells. No fluorescence signal could be observed in the Annexin V-cy3 channel or the D 3 fluorescein channel, confirming that all cells were healthy over the period of incubation, and that D 3 loading did not induce apoptosis ( Fig. 1b ). When the cells were treated with an apoptosis inducer, staurosporine (SSP), for 4 h, the FITC fluorescence signal of D 3 was found co-existing with the Annexin V-cy3 apoptosis signal ( Fig. 1c ). The FITC fluorescence intensity of cell lysates of the SSP-treated cells was threefold higher than that of the cells without SSP, or the unlabelled cells ( Fig. 1d ). Similar results were also found in HeLa cells. To confirm that PDL degradation is a possible mechanism of fluorescence increase in D 3 -treated cells, cell lysates were collected and ran through a size-exclusion column. The fluorescence of each collected fraction was measured. High fluorescence was observed in the low-molecular-weight fractions, thereby suggesting that PDL was degraded during apoptosis ( Fig. 1e ). These data support the hypothesis that D 3 activation is apoptosis dependent. 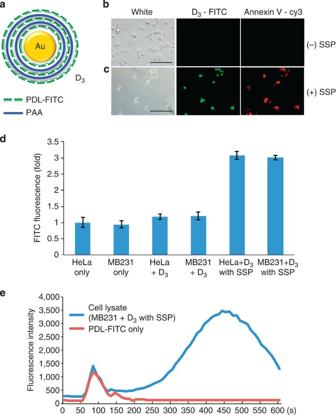Figure 1: Activation of D3nanoprobes after apoptosis induction in various cells. (a) Schematic diagram of D3. (b) MDA-MB231 cells incubated with D3or Annexin V-cy3 were imaged without or (c) with apoptosis induction using SSP (4 μM) for 4 h. Fluorescence signals were assessed using fluorescence microscopy (magnification: × 40). Scale bar, 100 μm. (d) D3was incubated with or without apoptosis induction in HeLa and MDA-MB231 cells, and FITC fluorescence intensity in cell lysates was examined. The fluorescence intensity of HeLa cells without treatment was set as onefold. Each experiment was done in triplicate and the data were shown as mean fluorescence±s.d. (e) Free PDL–FITC or the collected cell lysate from D3-labelled and SSP-treated cells was separated by size-exclusion chromatography. The FITC fluorescence intensity of each fraction was plotted. Note that the broad fluorescence peak at later time points indicated low-molecular-weight degraded fragments of PDL. Figure 1: Activation of D 3 nanoprobes after apoptosis induction in various cells. ( a ) Schematic diagram of D 3 . ( b ) MDA-MB231 cells incubated with D 3 or Annexin V-cy3 were imaged without or ( c ) with apoptosis induction using SSP (4 μM) for 4 h. Fluorescence signals were assessed using fluorescence microscopy (magnification: × 40). Scale bar, 100 μm. ( d ) D 3 was incubated with or without apoptosis induction in HeLa and MDA-MB231 cells, and FITC fluorescence intensity in cell lysates was examined. The fluorescence intensity of HeLa cells without treatment was set as onefold. Each experiment was done in triplicate and the data were shown as mean fluorescence±s.d. ( e ) Free PDL–FITC or the collected cell lysate from D 3 -labelled and SSP-treated cells was separated by size-exclusion chromatography. The FITC fluorescence intensity of each fraction was plotted. Note that the broad fluorescence peak at later time points indicated low-molecular-weight degraded fragments of PDL. Full size image Cell fate tracker from live to dead (DL 2 ) Based on these observations, the original nanoparticle was re-designed to carry two reporters, one for the healthy stage and a second for the dying stage. AuNPs were first coated with PDL–FITC (D), spaced by a layer of counter ion polymer PAA (DA) and then followed by PLL-C6 (DL), PAA (DLA) and PLL-C6 (DL 2 ). The assembled DL 2 particle has one inner layer of PDL–FITC and two layers of PLL-C6, separated by two layers of PAA using electrostatic interactions ( Fig. 2a ). The hydrodynamic diameter of the prepared nanoprobes was measured by dynamic light scattering after coating with each layer. The size of the initial bare AuNPs was 40 nm and the prepared particle size increased steadily with the number of layers (D: 54 nm; DL: 87 nm; DL 2 : 113 nm; Fig. 2b ). The alternating layers of charged polyelectrolytes were evidenced by the zigzag pattern of the surface zeta potentials ( Fig. 2b ). The PLL and PDL layers converted the surface charge from negative to positive, whereas the PAA layers converted the surface charge from positive to negative. 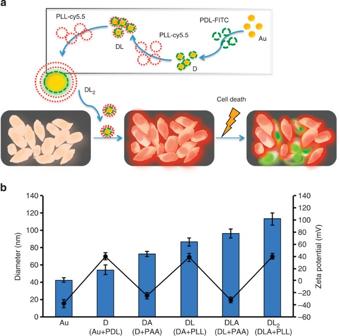Figure 2: Preparation of cell fate tracker DL2. (a) Schematic illustrating the process of preparing multilayered nanoprobes using PDL–FITC/PLL-cy5.5 and PAA as the charged polyelectrolytes. Negatively charged PAA layers that are placed between PDL–FITC and/or PLL-cy5.5 layers are omitted from the illustration for simplicity. (b) The average size (blue bar) and zeta potential (black circle) of each multilayered nanoprobe. All measurements were done in triplicate and the data were shown as mean±s.d. Figure 2: Preparation of cell fate tracker DL 2 . ( a ) Schematic illustrating the process of preparing multilayered nanoprobes using PDL–FITC/PLL-cy5.5 and PAA as the charged polyelectrolytes. Negatively charged PAA layers that are placed between PDL–FITC and/or PLL-cy5.5 layers are omitted from the illustration for simplicity. ( b ) The average size (blue bar) and zeta potential (black circle) of each multilayered nanoprobe. All measurements were done in triplicate and the data were shown as mean±s.d. Full size image To demonstrate the usage of this all-in-one probe, MDA-MB231 cells were labelled with DL 2 . After the excess particles were washed away, the cells were cultured in normal culture medium and monitored under a fluorescence microscope daily. As previously observed, the PLL layers of the internalized DL 2 were activated by normal intracellular proteolysis and produced a stable and long-lasting cy5.5 signal. During a 4-day incubation, no fluorescein signal, indicating apoptosis, was detected ( Fig. 3a ). When the apoptosis inducer SSP was added to the culture medium on day 4, cell death was incurred and, in consequence, green fluorescein signal was generated ( Fig. 3b ). These data strongly suggest that DL 2 is suitable for long-term cell labelling and does not produce false apoptotic signals, because under normal conditions healthy cells do not hydrolyse or activate the PDL molecule. Once apoptosis occurred, the PDL layer was degraded and the death signal was activated. A positive apoptosis control using a D 3 nanoprobe gave only an FITC signal, but no cy5.5 signals in cells ( Fig. 3b ). 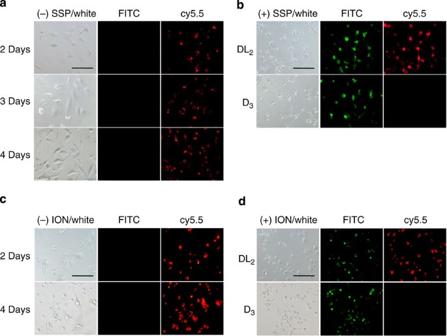Figure 3: Live- and dead-cell imaging with DL2in MDA-MB231 cells. (a,c) After incubation for 12 h with DL2(or D3), fluorescence signals were assessed by fluorescence microscopy for 4 days. (b,d) After 4 days, cells were incubated with SSP (4 μM) for 4 h to induce apoptosis (b) or ionomycin (ION, 10 μM) for 4 h to induce necrosis (d). Fluorescence signals mediated by DL2or D3were assessed in FITC and cy5.5 channels. Scale bar, 100 μm. Figure 3: Live- and dead-cell imaging with DL 2 in MDA-MB231 cells. ( a , c ) After incubation for 12 h with DL 2 (or D 3 ), fluorescence signals were assessed by fluorescence microscopy for 4 days. ( b , d ) After 4 days, cells were incubated with SSP (4 μM) for 4 h to induce apoptosis ( b ) or ionomycin (ION, 10 μM) for 4 h to induce necrosis ( d ). Fluorescence signals mediated by DL 2 or D 3 were assessed in FITC and cy5.5 channels. Scale bar, 100 μm. Full size image It is known that apoptosis is not the sole pathway causing cell death; necrosis also occurs under many conditions. To evaluate the potential usage of a PDL-containing nanoprobe in necrosis imaging, MDA-MB231 cells were incubated with DL 2 and then treated with a widely used necrosis inducer, ionomycin [34] . As seen in Fig. 3c,d , the necrotic cells fluoresced after induction, suggesting that PDL was also degraded during necrosis. Human mesenchymal stem cells tracking To test the feasibility of the nanoprobe in tracking therapeutic cells in vitro and in vivo , human mesenchymal stem cells (hMSCs) were first incubated with DL 2 and imaged before and after apoptosis induction. As previously observed in MDA-MB231 cancer cells, only the life signal of cy5.5 were generated in all hMSCs over a 4-day period. No FITC death signal was detected in hMSCs ( Fig. 4a ), until the apoptosis inducer SSP was added to the medium ( Fig. 4b ). Following the in vitro tracking confirming imaging result, DL 2 was tested in tracking hMSCs in vivo . DL 2 -labelled hMSCs were injected directly into the mouse ear pinna and then the mice were imaged using a home-built confocal microscopy [35] . In 2 h, the majority of the cells maintained their viability by cy5.5 expression ( Fig. 4c ). However, a small portion of the injected cells showed evidence of cell death by labelling with FITC in addition to cy5.5. These results support the potential of DL 2 to label live and dead stem cell populations in vivo . 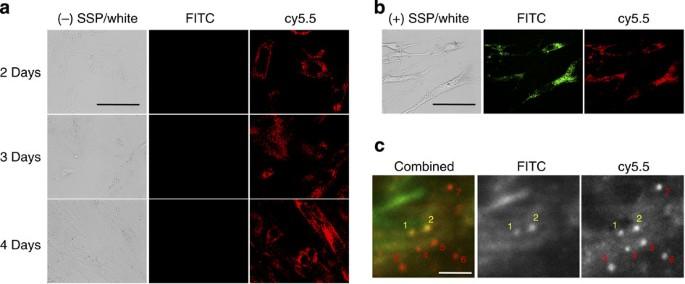Figure 4: Live- and dead-MSC imaging with DL2in vitroandin vivo. (a) After incubation hMSCs for 12 h with DL2, fluorescence signals were assessed by fluorescence microscopy for 4 days. Scale bar, 100 μm. (b) After 4 days, hMSCs were incubated with 4 μM of SSP for 4 h to induce cell apoptosis. Fluorescence signals mediated by DL2were assessed in each FITC and cy5.5 channels. Scale bar, 100 μm. (c) MSCs labelled with DL2could be visualizedin vivoafter local injection in the dermis of the mouse ear pinna. MSCs (1~7) labelled with DL2were strongly fluorescent in the cy5.5 channel. A small portion of the cells (1 and 2) were co-stained in the FITC channel, indicating that they were undergoing cell death. The signal-to-background ratio was 1.20 and 1.35 for cell 1 and cell 2, respectively. Scale bar, 50 μm. Figure 4: Live- and dead-MSC imaging with DL 2 in vitro and in vivo . ( a ) After incubation hMSCs for 12 h with DL 2 , fluorescence signals were assessed by fluorescence microscopy for 4 days. Scale bar, 100 μm. ( b ) After 4 days, hMSCs were incubated with 4 μM of SSP for 4 h to induce cell apoptosis. Fluorescence signals mediated by DL 2 were assessed in each FITC and cy5.5 channels. Scale bar, 100 μm. ( c ) MSCs labelled with DL 2 could be visualized in vivo after local injection in the dermis of the mouse ear pinna. MSCs (1~7) labelled with DL 2 were strongly fluorescent in the cy5.5 channel. A small portion of the cells (1 and 2) were co-stained in the FITC channel, indicating that they were undergoing cell death. The signal-to-background ratio was 1.20 and 1.35 for cell 1 and cell 2, respectively. Scale bar, 50 μm. Full size image A cytotoxicity assay of the prepared nanoprobes showed no significant cytotoxicity in MDA-MB231, HeLa or hMSCs after treatment with various nanoprobes for 24 h ( Supplementary Fig. 4 ). Death signal and reactive oxygen species The cultured results indicated that PDL is stable in healthy cells for long periods of time, but broken down quickly during apoptosis or necrosis. It is known that proteases recognize L -form amino acid residues and degrade L -peptides with efficiency. In contrast, D -form amino acid residues cannot be recognized by most proteases; thus, D -amino acid-capped peptides or -formed peptides have been proposed to prolong the blood half-life of peptide drugs or peptide-based delivery systems [36] . There is little literature report about the biodegradation of D -peptides, besides an early report of PDL hydrolysis by pancreatic enzyme extracts [37] . A better understanding of the possible mechanism for PDL degradation is tempting. Among the common factors that participate in cell death, reactive oxygen species (ROS) play critical roles in inducing apoptosis and necrosis [38] , [39] , [40] , [41] . In addition, mounting evidence supports that SSP increases ROS production and induces cell death by promoting the intrinsic apoptotic pathway [42] , [43] , [44] , [45] . As cellular oxidative stress results from the increased ROS, and thus is directly linked to the induction of cell death [46] , it is thus suspected that ROS could contribute to PDL degradation. To verify this hypothesis, a ROS scavenger, N-acetylcysteine amide (NACA) [47] , [48] , was used to quench ROS in cell culture. MDA-MB231 cells were pretreated with NACA for 30 min before the apoptosis induction with SSP (4 μM) for 2 h. The production of ROS induced by SSP was increased by twofold, as compared with the untreated control ( Fig. 5a ), while the NACA pretreatment was able to lower ROS production to the baseline level. Interestingly, the FITC death signal caused by SSP-induced apoptosis was also diminished, as NACA was included in the DL 2 -labelled MDA-MB231 cells, thus suggesting that ROS production could be involved in PDL degradation ( Fig. 5b ). 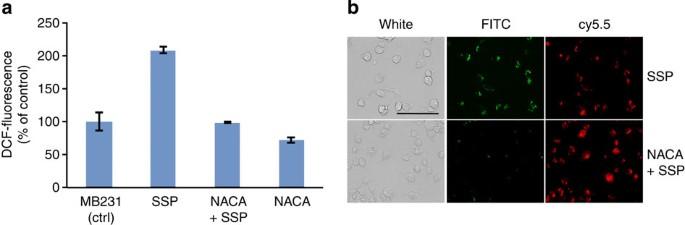Figure 5: Correlation between ROS production and cell death signal. (a) DCF fluorescence intensity was measured after treating MDA-MB231 cells with SSP (4 μM) for 2 h in the presence or absence of NACA (1 mM). The fluorescence intensity of the untreated MDA-MB231 cells was set as 100%. Each experiment was performed at least three times and the results were expressed as the median change in fluorescence±s.d. (b) Fluorescence images of DL2-incubated MDA-MB231 cells after apoptosis induction with SSP (4 μM, 2 h) in the presence or absence of NACA (1 mM). The FITC signal was significantly reduced in the NACA-treated cells. Scale bar, 100 μm. Figure 5: Correlation between ROS production and cell death signal. ( a ) DCF fluorescence intensity was measured after treating MDA-MB231 cells with SSP (4 μM) for 2 h in the presence or absence of NACA (1 mM). The fluorescence intensity of the untreated MDA-MB231 cells was set as 100%. Each experiment was performed at least three times and the results were expressed as the median change in fluorescence±s.d. ( b ) Fluorescence images of DL 2 -incubated MDA-MB231 cells after apoptosis induction with SSP (4 μM, 2 h) in the presence or absence of NACA (1 mM). The FITC signal was significantly reduced in the NACA-treated cells. Scale bar, 100 μm. Full size image ROS are active signalling molecules that direct the cell’s response to stress [49] , [50] . Under the extreme stress condition, such as apoptosis or necrosis, ROS initiate a chain of intracellular reactions, resulting in dramatic changes in the dynamic of hydrolysis [45] . PDL could be hydrolysed quickly when it was exposed to this stimulated environment. Besides, if PDL and ROS are in close contact, ROS may cause direct chemical fragmentation. It is clear that more systematic cellular studies with all types of ROS are required to elucidate the detailed molecular mechanism of PDL activation. In summary, a chameleon-like multilayered nanoprobe was successfully fabricated by layer-by-layer deposition. The nanoprobe was taken up efficiently and showed vital fluorescence signal immediately in live cells. This PLL fluorescence persisted for long periods of time due to the tight coating of the layers and the slow release of the degraded fluorescent signal [30] . As cells began dying, a different fluorescence signal was turned on. The death signal was caused by the degradation of PDL, presumably induced by robust ROS production during either the apoptotic or necrotic death process. However, the detail mechanism of ROS-induced PDL degradation remains to be elucidated. The in vivo feasibility study demonstrated the potential of studying implanted therapeutic cells in real time. The vital status of cells, whether they are live or dead, can be identified clearly by their fluorescence colour. This study provides a well-defined nanoprobe with the unique property of long-term cell tracking. Materials PLL (molecular weight (Mw)=30,000~70,000 Da), PDL (Mw=30,000~70,000 Da), PAA (35 wt.% solution, average Mw=15,000 Da), FITC, SSP, Annexin V-cy3, ionomycin and NACA were obtained from Sigma-Aldrich (St Louis, MO). Bare AuNPs (40 nm) were purchased from BB International (Cardiff, UK), Sephadex G-50 was from GE Healthcare Bio-Sciences (Pittsburgh, PA), Amicon Ultracel membrane (10 kDa) was from Millipore (Billerica, MA), CellTiter aqueous one solution was from Promega (Madison, WI) and DCFDA Cellular ROS Detection Assay Kit was from Abcam (Cambridge, MA). Preparation and validation of PLL-cy5.5 Various amounts of cy5.5 (0.0125, 0.025, 0.05, 0.1 or 0.2 mg) in water (100 μl) were reacted with PLL (0.2 mg) in NaHCO 3 (1 mM, 100 μl) in the dark at room temperature for 30 min (vortexed every 10 min). The reaction products were separated using molecular weight cutoff membrane filters (10 kDa, Millipore). The resulting PLL-cy5.5 with different loads were collected and washed several times with sterilized water until the colour of the filtrate was clear. The loading ratio of cy5.5 per PLL was calculated based on the absorbance of cy5.5. The cy5.5/PLL ratios were from 1/1 (PLL-C1) to 7/1 (PLL-C7) as the amount of cy5.5 was increased. The prepared PLL-cy5.5 (PLL 0.2 nmol in 5 μl) with various loads of cy5.5 were incubated with trypsin–EDTA (10 μl, 0.25%, Sigma-Aldrich) in PBS (185 μl) in a 96-well culture plate at 37 °C. The increase in cy5.5 fluorescence signal caused by dequenching was assessed using a plate reader (Tecan, Männedorf, Switzerland) with 665 nm excitation and 700 nm emission for 15 h. Preparation of PDL–FITC FITC (0.4 mg) in dimethylformamide solution (500 μl) was reacted with PDL (0.2 mg) in NaHCO 3 (1 mM, 500 μl), with constant shaking in the dark at room temperature for 2 h. The reaction products were separated using molecular weight cutoff membrane filters (10 kDa, Millipore). The resulting PDL–FITC was collected and washed several times with sterilized water until the colour of filtrate was clear. The loading ratio of FITC per PDL was 6/1, as calculated based on the absorbance of FITC. Preparation and characterization of multilayered nanoprobe All nanoprobes were prepared using the same protocol, except the deposition of PLL or PDL layers. DL 2 is described in detail here. Based on previously developed protocols [30] , [51] , [52] , a AuNP solution (40 nm, 3.15 × 10 9 particles in 700 μl) was added dropwise to a PDL–FITC solution (PDL, 1.8 nmol in 500 μl). After gentle shaking in the dark for 30 min, the solution was centrifuged (30 min at 16,100 g ) using a microcentrifuge (Eppendorf, Hauppauge, NY). The supernatant was removed and the gel-like deep red pellet was resuspended in pure water and centrifuged again (30 min at 16,100 g ). After another wash, PDL–FITC-coated AuNPs were re-suspended in pure water (500 μl). Next, the PDL–FITC-coated AuNPs were added to a PAA solution (23.3 mM, 500 μl). The reaction solution was incubated in the dark for 30 min with gentle shaking, followed by three washes. The deposition procedures were repeated with PLL-C6, instead of PDL–FITC, and PAA to have five layers of polyelectrolyte (one layer of PDL–FITC, two layers of PLL-cy5.5 and two layers of PAA). Sizes and zeta potentials of the prepared nanoparticles in water were measured using Zeta-PALS apparatus (Brookhaven, Holtsville, NY) according to the manufacturer’s instructions. D 3 and L 3 were prepared in the same manner but using only PDL–FITC or PLL-C6, respectively. Protease-assisted fluorescence release from L 3 The protease-sensitivity of various PLL-cy5.5-coated AuNPs (three layers) was determined by incubating the particles (7.88 × 10 8 particles) in a 96-well culture plate with or without trypsin (25 μl) in PBS at 37 °C. The increase in the cy5.5 fluorescence signal was analysed using a plate reader (Tecan) at 665 nm excitation and 700 nm emission for 24 h. Cell lines MDA-MB231 human breast cancer cells and HeLa cells were purchased from ATCC (Manassas, VA) and cultured in DMEM medium (Mediatech Inc., Manassas, VA) supplemented with 2 mM L -glutamine, 100 U ml −1 penicillin, 100 mg ml −1 streptomycin and 10% heat-inactivated fetal bovine serum (Sigma-Aldrich). hMSCs were obtained from Lonza (Walkersville, MD) and cultured in growth medium (Mesenchymal Stem Cell Growth Medium Bullet Kit, Lonza). hMSCs between the third and fifth passage were used for all experiments. All cells were cultured in a humidified atmosphere with 5% CO 2 at 37 °C. Apoptosis imaging with D 3 and Annexin V-cy3 MDA-MB231 cells were collected by trypsinization, counted and plated in a 96-well black clear-bottom culture plate (Corning, Pittston, PA) at a density of 1 × 10 3 cells per well. After 1 day, D 3 nanoparticles (2.52 × 10 8 particles) were added and incubated for 12 h. Cells were then washed three times with PBS and cultured in phenol red-free medium. At the indicated time points, cells were treated with or without SSP (4 μM, 4 h, 37 °C) and then stained with Annexin V-cy3 (10 ng) for 15 min at 37 °C. After washing with PBS, cells were imaged under a fluorescence microscope (Olympus, Tokyo, Japan). Quantitation of fluorescent signal changes in cell lysates MDA-MB231 cells and HeLa cells were seeded in a six-well culture plate (BD Falcon) at a density of 2 × 10 5 cells per well. One day later, D 3 nanoparticles (1.58 × 10 9 particles) were added to each well and cultured for additional 24 h. Cells were treated with SSP (4 μM) for 4 h at 37 °C to induce apoptosis. Cells were harvested, pelleted cells were lysed with 1 × lysis buffer (50 mM HEPES, pH 7.4, 5 mM CHAPS, 5 mM dithiothreitol) and the lysates were transferred to a 96-well black clear-bottom culture plate (Corning) and incubated for 3 h at 37 °C. The lysates were concentrated using a 10-kDa cutoff membrane (Millipore). The increase in the FITC fluorescence signal was assessed for 3 h at 37 °C using a plate reader (Tecan), with 480 nm excitation and 530 nm emission. PDL–FITC degradation by size-exclusion chromatography Sephadex G-50 (1.3 g) was swollen and equilibrated with 40 ml of PBS buffer for 2 h. Columns (1 cm × 30 cm) were packed to a final height of ~20 cm and eluted with at least one column volume of PBS before the addition of sample. Free PDL–FITC (FITC/PDL=6/1, PDL 0.2 nmol in 150 μl) or lysate of D 3 -labelled and SSP-treated (4 μM for 4 h) MDA-MB231 cells was applied to the equilibrated column and eluted at room temperature. Fractions were collected in eppendorf tubes after discarding the first 40 drops. Each elution tube contained eight drops, and the FITC fluorescence was measured using a plate reader (Tecan), with 480 nm excitation and 530 nm emission. Cell imaging of apoptosis and necrosis with D 3 and DL 2 MDA-MB231 cells were collected by trypsinization, counted and plated in a 96-well black clear-bottom culture plate (Corning) at a density of 2 × 10 3 cells per well. hMSCs were prepared the same, but at a density of 1 × 10 3 cells per well. After 1 day, D 3 or DL 2 nanoprobes (2.52 × 10 8 particles) were added and incubated for 12 h. Cells were washed three times with PBS, cultured in phenol red-free medium and, at the indicated time points, were treated with or without SSP (4 μM) or ionomycin (10 μM) for 4 h at 37 °C to induce apoptosis or necrosis, respectively. After washing with PBS, cells were imaged under a fluorescence microscope (Olympus). In vivo imaging of DL 2 -labelled hMSC After labelling hMSCs with DL 2 nanoprobes (9.45 × 10 8 particles) for 24 h in T-75 flask (Sigma-Aldrich), cells were collected and suspended at a concentration of 10 6 cells per ml. Around 10,000 cells (10 μl) were then intradermally injected into the ear pinna of three adult C57BL/6 mice (Charles River Laboratories, Wilmington, MA). The FITC and cy5.5 fluorescence of hMSCs in the ear were imaged using a home-built intravital confocal scanning microscope [35] . The studies were in accordance with US National Institutes of Health guidelines for care and use of animals under approval of the Institutional Animal Care and Use Committees of Massachusetts General Hospital and Harvard Medical School. Cytotoxicity assessment of the multilayered nanoprobes A cell proliferation assay was performed to assess the cytotoxicity of the various treatments. Briefly, MDA-MB231 cells, HeLa cells and hMSCs were collected by trypsinization, counted and plated in a 96-well culture plate at a density of 5 × 10 3 cells (or 2.5 × 10 3 of hMSCs) per well. One day after seeding, various nanoprobes (2.52 × 10 8 particles) were added and the cells were cultured for additional 24 h. At day 2, 20 μl CellTiter solution (Promega) was added to each well and incubated for 3 h. The absorbance of the solution was then measured at 490 nm using a plate reader (Tecan). Measurement of intracellular ROS The level of intracellular ROS was determined using a DCFDA (2′, 7′-dichlorofluorescein diacetate) Cellular ROS Detection Assay Kit (Abcam) according to the manufacturer’s instructions. Briefly, MDA-MB231 cells were collected by trypsinization, counted and plated in a 96-well black clear-bottom culture plate (Corning) at a density of 2 × 10 4 cells per well. After 1 day, cells were incubated with DCFDA (20 μM) for 45 min at 37 °C in the dark and then treated with or without 1 mM of NACA for 30 min. SSP (4 μM) in phenol red-free medium was added to induce apoptosis for 2 h. The level of ROS was determined by measuring the fluorescence intensity using a microplate reader (Tecan), with excitation at 485 nm and emission at 535 nm. Fluorescence change according to ROS production MDA-MB231 cells were collected by trypsinization, counted and plated in μ-Slide eight-well chambered cover slip (Ibidi, Martinsried, Germany) at a density of 5 × 10 3 cells per well. After 1 day, DL 2 nanoprobes (3.78 × 10 8 particles) were added and incubated for 12 h. The cells were then washed three times with PBS and cultured in phenol red-free medium with or without NACA (1 mM) for 30 min. The cells were treated with SSP (4 μM) and cultured for additional 2 h. After washing with PBS, cells were imaged under EVOS FL Auto Cell Imaging System (Life Technologies, Carlsbad, CA). How to cite this article : Lee, S. K. et al. An authentic imaging probe to track cell fate from beginning to end. Nat. Commun. 5:5216 doi: 10.1038/ncomms6216 (2014).